Imaging the nanoscale organization of peptidoglycan in livingLactococcus lactiscells Bacterial cell walls constitute the frontier between cells and their environment, and therefore have several key functions, such as supporting the internal turgor pressure of the cell, protecting the cytoplasm from the outer environment, imparting shape to the organism, functioning as a molecular sieve and controlling interfacial interactions, that is, molecular recognition, cell adhesion and aggregation [1] , [2] . Understanding these functions requires elucidation of the molecular architecture of bacterial cell walls. The wall mechanical strength in eubacteria is provided by peptidoglycan, a polymer that is made up of glycan strands that are crosslinked by peptide side chains [3] . In Gram-negative bacteria, a thin peptidoglycan layer is overlayed by an outer membrane, that is, an asymmetrical bilayer of phospholipids and lipopolysaccharides containing membrane proteins (for example, porins) [4] , whereas in Gram-positive bacteria, a thick layer of peptidoglycan constitutes the main body of the cell wall. Here, the peptidoglycan network is crossed by anionic polymers, mainly teichoic acids, which are bound to the cytoplasmic membrane (lipoteichoic acids) or to the peptidoglycan network itself (wall teichoic acids) [5] , [6] . An additional outer layer of cell wall (or exo) polysaccharides may sometimes be present. Besides its mechanical function, peptidoglycan is also the target of major classes of antibiotics, including β-lactams and glycopeptides. Despite the multiple important functional roles of peptidoglycan, its three-dimensional organization remains controversial [7] . In the classical model, glycan strands are believed to run parallel to the plasma membrane [8] , arranged perhaps as hoops or helices around the short axis of the cell, resulting in a woven fabric [9] . This model is supported by recent experimental data obtained on isolated sacculi from Gram-negative bacteria Escherichia coli and Caulobacter crescentus [10] , and from the rod-shaped Gram-positive bacterium Bacillus subtilis [11] . An alternative 'scaffold' model suggests that the strands are oriented vertically with respect to the membrane [12] , [13] . Hence, understanding the spatial arrangement of peptidoglycan is a challenging issue. In the past few years, atomic force microscopy (AFM) has been established as a powerful imaging technique in microbiology [14] , [15] , enabling us to visualize the nanoscale architecture of single live cells while they grow [16] , [17] or interact with drugs [18] , [19] , and to detect and localize single cell wall constituents [20] , [21] , [22] , [23] . In this study, we use AFM topographic and recognition imaging to explore the nanoscale organization of cell wall peptidoglycan in living Lactococcus lactis bacteria. The use of mutant strains impaired in the production of cell wall polysaccharides (WPS) [24] enables us to reveal the native architecture of cell wall peptidoglycan. Topographic images show 25-nm-wide periodic ridges on the mutant surface that always run parallel to the short cell axis. Recognition imaging demonstrates that these ridges are made of peptidoglycan. The results are consistent with a peptidoglycan organization in the plane perpendicular to the long axis of the cell. Topographic imaging of wild-type cells Bacteria were immobilized in porous polymer membranes, a method allowing AFM analysis of living cells while preserving their native macromolecular architecture [25] . 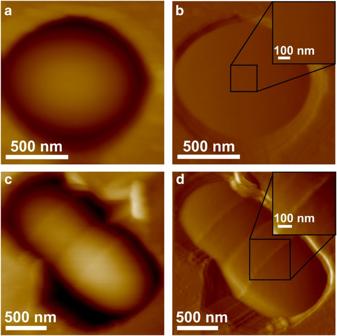Figure 1: AFM images of WTL. lactiscells. (a,c) Height and (b,d) deflection images recorded in sodium acetate buffer forL. lactisWT cells using a small applied force (250 pN). The images show either the pole of a single cell (a,b) or two cells during the course of the division process (c,d). Insets inbanddshow high-resolution deflection images recorded in the square regions. Figure 1 shows height and deflection images of L. lactis wild-type (WT) cells. Because of the large curvature of the cells, height images ( Fig. 1a,c ) had a fairly poor resolution, whereas deflection images ( Fig. 1b,d ) were much more sensitive to the fine surface relief. The polar region observed at small imaging forces ( ∼ 250 pN) was very smooth and did not show any peculiar topographic feature ( Fig. 1b ). Dividing cells were also smooth but showed well-defined division septum, as well as ring-like structures at a certain distance from the septum ( Fig. 1d ). These annular structures, presumably formed by an outgrowth of the cell wall, are similar to the so-called 'equatorial rings' in streptococci, which mark the position of the division site, duplicate and then separate to form the edges of the newly synthesized peptidoglycan zone during cell elongation [26] . These structural features are in agreement with previous AFM observations [21] , [22] . Figure 1: AFM images of WT L. lactis cells. ( a , c ) Height and ( b , d ) deflection images recorded in sodium acetate buffer for L. lactis WT cells using a small applied force (250 pN). The images show either the pole of a single cell ( a , b ) or two cells during the course of the division process ( c , d ). Insets in b and d show high-resolution deflection images recorded in the square regions. Full size image It is noteworthy that major differences in surface structure were observed when imaging cells at large imaging forces ( ∼ 5 nN). 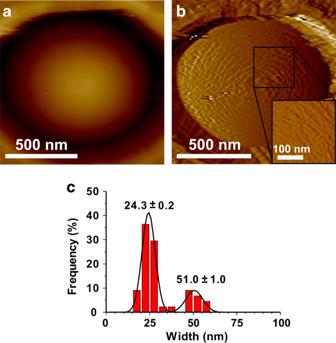Figure 2: Imaging WT cells at large forces causes substantial ultrastructural changes. (a) Height and (b) deflection images of the polar region of anL. lactisWT cell recorded with an applied force of 5 nN. The inset shows a high-resolution deflection image recorded in the square region. (c) Statistical analysis of the width of the periodic features observed in height images (n=45 measurements on two different cells, average width ± s.e.m.). As can be seen in Figure 2 , the cell pole was rougher and showed concentric striations separated by 25 and 50 nm, which are reminiscent of features observed earlier on Staphylococcus aureus cells by AFM [19] , [27] and electron microscopy [28] , [29] , [30] . We suggest that these ring-like structures reflect 25-nm-wide peptidoglycan bands of the L. lactis cell wall, a hypothesis that is directly supported by our single-molecule recognition data (see below). The observation of 50-nm-wide rings would therefore reflect double bands that could not be resolved individually because of finite tip geometry (tip radius ∼ 25 nm). As pointed out by Touhami et al . [27] , the concentricity of rings implies that peptidoglycan strands are, themselves, oriented in a similar manner and are added or removed in an orderly manner. We note that, as opposed to the S. aureus situation, peptidoglycan strands were never seen when imaging L. lactis at small forces. Consistent with electron microscopy observations, [24] and with our previous research [22] , this indicates that in WT L. lactis , peptidoglycan is covered by an outer layer of cell surface constituents, mainly cell WPS. Figure 2: Imaging WT cells at large forces causes substantial ultrastructural changes. ( a ) Height and ( b ) deflection images of the polar region of an L. lactis WT cell recorded with an applied force of 5 nN. The inset shows a high-resolution deflection image recorded in the square region. ( c ) Statistical analysis of the width of the periodic features observed in height images ( n =45 measurements on two different cells, average width ± s.e.m.). Full size image Topographic imaging of cell wall mutants To further investigate whether peptidoglycan is indeed hidden by cell surface polymers, we analysed L. lactis mutants VES5748 and VES5751, which carry point mutations in the operon encoding the synthesis of cell WPS [24] . We first confirmed that the outermost surface composition of WPS − mutants is poorer in polysaccharides using X-ray photoelectron spectroscopy (XPS) [31] , [32] . Consistent with the general biochemical composition of bacterial cell walls, the main elements that were detected were C 1s , O 1s and N 1s ( Table 1 ). Sulphur, usually found in proteins in the form of cysteines and methionines, was never detected (<0.1%), whereas phosphorus, which is abundant in teichoic acids, was present in very small amounts (<1%). The validity of the XPS analysis was supported by two observations: (i) data for the WT strain were very similar to those previously obtained on a similar L. lactis strain [33] ; (ii) the two WPS − mutants showed very similar surface chemical compositions. To gain a biomolecular view of the cell surface, XPS data were converted into concentrations of basic model compounds [34] , namely, peptides, glycans and lipids ( Table 1 ). This modelling approach was previously validated in Gram-positive bacteria by correlating XPS and biochemical data obtained on various strains [34] . Assuming that peptidoglycan consists approximately of 50% glycans and 50% peptides [34] , we found that the data for the two WPS − mutants were consistent with a peptidoglycan surface, together with some lipids. By contrast, the WT strain was much richer in glycans than in peptides, indicating that, besides peptidoglycan, polysaccharides were also present in large amounts at the surface. This agrees well with electron microscopy data showing that in the WT, but not in WPS − mutants, cell wall peptidoglycan is covered by a thin layer of polysaccharides [24] . It is to be noted that, besides peptidoglycan and polysaccharides, teichoic acids and proteins are likely to be present as well. Yet, the lack of sulphur (<0.1%) and the very small amount of phosphorus (<1%) suggests that they are exposed only in small amounts. Hence, XPS revealed that the outermost surface of WPS − mutants is essentially composed of peptidoglycan. Table 1 Surface chemical composition measured by XPS, and proportions of carbon involved in peptides (C Pe ), glycans (C Gl ) and lipids (C Lp ) deduced from the data. Full size table We therefore postulated that WPS − mutants should expose naked peptidoglycan directly visible by AFM. 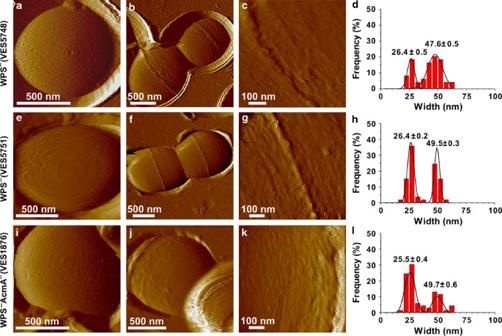Figure 3: AFM images of mutant strains reveal periodic bands running parallel to the short cell axis. Deflection images of polar regions (a,e,i) and of dividing bacteria (b,c,f,g,j,k) recorded forL. lactisVES5748 (a–c) and VES5751 (e–g) WPS−mutants lacking cell wall exopolysaccharides, and for the double mutant VES1876 WPS−AcmA−lacking both exopolysaccharides and the major autolysin AcmA (i–k). (c,g,k) High-resolution images obtained on the longitudinal region of the cells. All images were recorded in sodium acetate buffer using a small applied force (250 pN). (d,h,i) Statistical analysis of the width of the periodic features observed in the height images of VES5748 WPS−mutant (d,n=55 measurements, on five different cells), of VES5751 WPS−mutant (h,n=53 measurements, on four different cells, average width ± s.e.m.) and of VES1876 WPS−AcmA−double mutant (i,n=57 measurements, on three different cells, average width ± s.e.m.). Indeed, Figure 3 shows that the cell poles of both WPS − mutants imaged at small forces were much rougher than those of WT under similar conditions ( Fig. 1 ), and were decorated with 25-nm (50 nm)-wide concentric rings. Remarkably, ridges of similar width were also seen on the longitudinal region of the cells, and suggested the reflection of peptidoglycan bands running across the short axis of the cell. Unlike cocci such as S. aureus , which only exhibit septal division, ovococci such as L. lactis have an elongation phase as well [35] . Therefore, our finding that ridge structures are present over the entire cell surface indicates that they are not restricted to septation hydrolysis but are also observed in the elongation zone. These observations suggest that the lack of an outer layer of polysaccharides in WPS − mutants enables direct visualization of the peptidoglycan architecture. To obtain more quantitative information on surface roughness, we performed statistical analysis of height images at various scales of length. Root mean square roughness (R r.m.s. ) was analysed through the power spectral density of the fast Fourier transform of the height images [36] . It is noteworthy that major differences in roughness were observed when comparing WT and WPS − cells ( Supplementary Fig. S1 ). Although WT cells showed subnanometre roughness (R r.m.s. of 0.5 nm on 200×200 nm areas), WPS − cells were substantially rougher (R r.m.s. of ∼ 3 nm). We note that the increase in surface roughness correlates with electron microscopy observations revealing that mutations lead to the disappearance of an outer layer and to a more complex surface structure [24] . Figure 3: AFM images of mutant strains reveal periodic bands running parallel to the short cell axis. Deflection images of polar regions ( a , e , i ) and of dividing bacteria ( b , c , f , g , j , k ) recorded for L. lactis VES5748 ( a – c ) and VES5751 ( e – g ) WPS − mutants lacking cell wall exopolysaccharides, and for the double mutant VES1876 WPS − AcmA − lacking both exopolysaccharides and the major autolysin AcmA ( i – k ). ( c , g , k ) High-resolution images obtained on the longitudinal region of the cells. All images were recorded in sodium acetate buffer using a small applied force (250 pN). ( d , h , i ) Statistical analysis of the width of the periodic features observed in the height images of VES5748 WPS − mutant ( d , n =55 measurements, on five different cells), of VES5751 WPS − mutant ( h , n =53 measurements, on four different cells, average width ± s.e.m.) and of VES1876 WPS − AcmA − double mutant ( i , n =57 measurements, on three different cells, average width ± s.e.m.). Full size image Do the observed ridges reflect artifactual hydrolysis activity caused by experimental conditions or are they an intrinsic feature of the cell wall? To tackle this problem, we first analysed the surface of a double mutant WPS − AcmA − , which lacks both cell WPS and the major autolysin AcmA. AcmA is the major autolysin ( N -actyl-glucosaminidase) of L. lactis that is responsible for cell autolysis in the stationary phase [37] , [38] . The AcmA − mutant is only deficient in final cell separation and not in division, indicating that it is clearly viable [37] . Autolysis assays in the presence of Triton X-100 indeed confirmed that AcmA − and WPS − AcmA − mutant cells have strongly reduced hydrolysis activity, compared with WT cells ( Supplementary Fig. S2 ). As can be seen in Figure 3i–l , double mutant WPS − AcmA − displayed striations or ridges with 25 nm periodicity that were very similar to those seen in WPS − mutants. Second, we analysed the VES5748 WPS − mutant in phosphate buffer, which, unlike sodium acetate buffer, does not prevent hydrolysis ( Supplementary Fig. S2 ). We found that even after 2 h the cells still featured well-defined 25-nm-spaced ridges similar to those observed in sodium acetate buffer ( Supplementary Fig. S3 ). The same observation could be made for cells resuspended in ultrapure water for 2 h or in sodium acetate buffer for 10 h. These data indicate that the ridges were reproducibly observed in very different environmental conditions, thus consistent with the notion that they are an intrinsic feature of the cell wall. Another interesting issue is whether ridge structures are still observed on purified sacculi. To approach this question, we imaged, in air, gently broken peptidoglycan sacculi from the L. lactis VES5748 mutant ( Fig. 4 ). From the double wall thickness ( ∼ 40 nm), we estimated the average single wall thickness to be ∼ 20 nm. We note that this single cell wall thickness of 20 nm measured in air is compatible with hydrated cables of 25 nm diameter. The 5 nm difference could result from various factors, including shrinkage of the structures on dehydration, and erosion by chemical and enzymatic treatments. Ring-like structures, presumably reflecting the equatorial rings, were still observed on the outer wall surface ( Fig. 4a–c ). However, parallel ridges were no longer seen ( Fig. 4d ), neither on the outer surface nor on the inner surface, indicating that these architectural features can only be observed on live cells. Our finding that parallel bands are missing in sacculi could be due to many factors, such as the lack of high internal osmotic pressure and the removal of peptidoglycan-associated polymers. These data emphasize the importance of probing the peptidoglycan organization directly on live cells rather than on isolated structures that have been subjected to aggressive chemical and biological treatments. 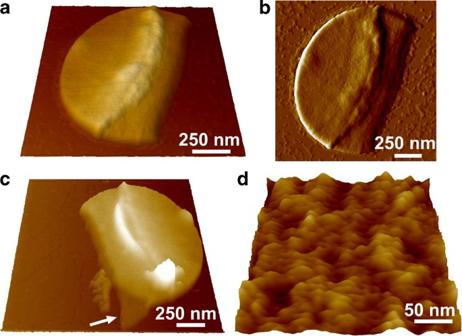Figure 4: Sacculi do not show parallel bands. (a,c,d) Height and (b) deflection images in air of peptidoglycan sacculi fromL. lactisVES5748, gently broken by a french press. Imagesaandbshow the outside surface of the same sacculus consisting of a double cell wall. Imagecrepresents another sacculus in which the boarder exposes the inner surface of a single wall (arrow). (d) High-resolution view of the outer surface, similar morphology being observed on the inner surface. Figure 4: Sacculi do not show parallel bands. ( a , c , d ) Height and ( b ) deflection images in air of peptidoglycan sacculi from L. lactis VES5748, gently broken by a french press. Images a and b show the outside surface of the same sacculus consisting of a double cell wall. Image c represents another sacculus in which the boarder exposes the inner surface of a single wall (arrow). ( d ) High-resolution view of the outer surface, similar morphology being observed on the inner surface. Full size image Single-molecule recognition imaging of peptidoglycan As a complementary approach to topographic imaging, we used recognition imaging to detect and localize individual peptidoglycan molecules on the different strains. To this end, spatially resolved force curves were recorded across the cell surface using AFM tips modified with the Lysin Motif (LysM) from the major autolysin AcmA, a protein module that specifically binds peptidoglycan [22] . 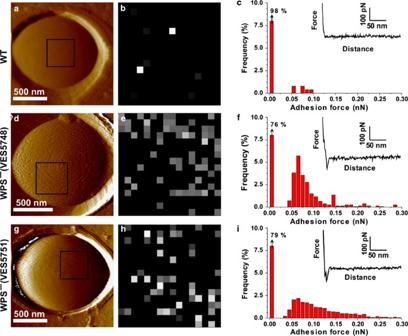Figure 5: Single-molecule recognition imaging of peptidoglycan. (a,d,g) Deflection images recorded with silicon nitride tips onL. lactisWT (a), VES5748 WPS−mutant (d) and VES5751 WPS−mutant (g). (b,e,h) Adhesion force maps (400×400 nm) recorded on the three strains with LysM tips in the square areas shown in the deflection images, using a maximum applied force of 250 pN. (c,f,i) Adhesion histograms generated from four adhesion force maps (n=1,024 curves), together with representative force curves. Figure 5a–c shows the adhesion (or recognition) map, adhesion histogram and typical force curve obtained on WT cells with an LysM-tip at low applied forces (250 pN). Most force curves did not show any binding events. Consistent with previous work [22] and with the above ultrastructural data, this observation confirms that peptidoglycan is hidden by other cell wall constituents. Figure 5: Single-molecule recognition imaging of peptidoglycan. ( a , d , g ) Deflection images recorded with silicon nitride tips on L. lactis WT ( a ), VES5748 WPS − mutant ( d ) and VES5751 WPS − mutant ( g ). ( b , e , h ) Adhesion force maps (400×400 nm) recorded on the three strains with LysM tips in the square areas shown in the deflection images, using a maximum applied force of 250 pN. ( c , f , i ) Adhesion histograms generated from four adhesion force maps ( n =1,024 curves), together with representative force curves. Full size image The VES5748 WPS − mutant showed a very different behaviour in that a substantial fraction of curves showed binding forces, yielding a mean adhesion frequency of 24 ± 5% ( Fig. 5d–f ). The observed force distribution showed a single well-pronounced maximum at 71 ± 16 pN. Several observations support the notion that the 71 pN binding force reflects the rupture of specific LysM–peptidoglycan complexes. First, the specificity of the interaction was confirmed by showing a dramatic reduction of adhesion frequency when performing the same experiment with a silicon nitride tip ( Supplementary Fig. S4a–c ; adhesion frequency=2 ± 2%) or in a solution containing 10 μg ml −1 of peptidoglycan ( Supplementary Fig. S4d–f ; adhesion frequency=3 ± 1%). Second, our measured binding force is close to the forces observed earlier on both purified peptidoglycan and L. lactis cells treated with trichloroacetic acid [22] . This leads us to conclude that peptidoglycan was detected on the mutant surface, consistent with the absence of an external polysaccharide layer. Similar conclusions could be drawn from the analysis of the VES5751 WPS − mutant ( Fig. 5g–i ), except that binding forces in the 100–200 pN range were more frequently observed, suggesting that the simultaneous detection of two or three molecules was more frequent. What is the spatial arrangement of peptidoglycan molecules on mutant cells? Whereas low-resolution recognition maps (16×16 pixels) showed a somewhat random distribution of the detected molecules, maps obtained at higher resolution (32×32 pixels) on dividing cells showed heterogeneous, anisotropic arrangements of recognition events ( Fig. 6 ). Indeed, many of the detected molecules were arranged as lines running parallel to the short cell axis, thus having an orientation similar to that of the periodic bands (ridges) observed in topographic images. Rotating the cell by 90° resulted in a 90° rotation of both recognition lines and topographic bands ( Fig. 6c,d ). To confirm that the observed recognition lines were statistically significant, we calculated adjusted R 2 values for 10 different lines (shown in Fig. 6c,d ) and found that they were always in the 0.85–0.95 range, supporting the occurrence of peptidoglycan lines. By contrast, adjusted R 2 values obtained for lines randomly placed in other orientations were always in the 0.0–0.2 range. This correlation between structural and recognition images provides direct evidence that peptidoglycan localizes on the mutant surface in the form of parallel bands. 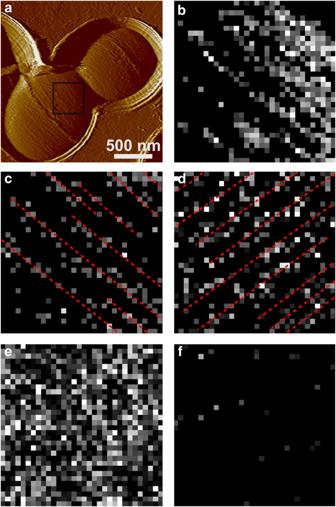Figure 6: Peptidoglycan localizes as parallel lines on the surface of WPS−mutants. (a) Deflection image of anL. lactisVES5748 WPS−mutant cell recorded with a silicon nitride tip. (b) Adhesion force map (400×400 nm) recorded with an LysM tip in the square area shown in the deflection image using a maximum applied force of 250 pN. (c–f) Adhesion force maps (500×500 nm) recorded with an LysM tip on another cell. Maps shown incanddwere recorded in the same area, except that the cell was rotated by 90°. Many of the detected molecules (bright pixels) were arranged as lines running parallel to the short cell axis (red lines). The map shown inewas obtained with a maximum applied force of 500 pN instead of 250 pN, whereas the map infwas obtained in a 10 μg ml−1peptidoglycan solution. In addition to the data shown, similar results were obtained in nine different cells from at least five different cultures, using 10 different tips from at least five different batches. Figure 6: Peptidoglycan localizes as parallel lines on the surface of WPS − mutants. ( a ) Deflection image of an L. lactis VES5748 WPS − mutant cell recorded with a silicon nitride tip. ( b ) Adhesion force map (400×400 nm) recorded with an LysM tip in the square area shown in the deflection image using a maximum applied force of 250 pN. ( c – f ) Adhesion force maps (500×500 nm) recorded with an LysM tip on another cell. Maps shown in c and d were recorded in the same area, except that the cell was rotated by 90°. Many of the detected molecules (bright pixels) were arranged as lines running parallel to the short cell axis (red lines). The map shown in e was obtained with a maximum applied force of 500 pN instead of 250 pN, whereas the map in f was obtained in a 10 μg ml −1 peptidoglycan solution. In addition to the data shown, similar results were obtained in nine different cells from at least five different cultures, using 10 different tips from at least five different batches. Full size image A pertinent question associated with the contrast of our recognition images ( Fig. 6 ) is why are there large areas of no interaction if peptidoglycan has been fully exposed in mutant strains? In single-molecule force spectroscopy experiments, it is known that binding frequency depends on the tip-sample contact area, a parameter that is influenced by several factors, among which are the maximum applied force and the sample surface geometry. We first verified whether our small applied force could explain the moderate binding frequency, by recording recognition maps on the VES5748 WPS − mutant using a force of 500 pN instead of 250 pN. Figure 6e clearly shows that this led to a marked increase in binding frequency, from 22 ± 5 to 68 ± 9%. This finding, which results from the increased contact area between the tip and the cell surface, supports the notion that peptidoglycan is a major constituent of the cell surface. In these high-force conditions, peptidoglycan lines can no longer be seen in the recognition maps ( Fig. 6e ), as they are essentially all in direct contact with each other. Here again, the specificity of the interaction was demonstrated by showing a dramatic reduction of the binding frequency after injection of a solution of peptidoglycan ( Fig. 6f ). Do cell surface geometry and roughness influence recognition contrast? As the radius of the tip apex is on the order of the width of the ridges ( ∼ 25 nm), it is tempting to suggest that, at small forces, peptidoglycan detection in between ridges is inhibited because of the tip shape. Therefore, we analysed VES5748 WPS − mutant cells that were boiled in the presence of trichloroacetic acid, a treatment known to alter the cell surface ultrastructure. Ridges were no longer observed in topographic images and the LysM tip was found to homogeneously bind to the surface using an applied force of 250 pN ( Supplementary Fig. S5 ). These observations lead us to believe that the peptidoglycan lines detected at low force correspond to the top of the topographic ridges. Another striking issue is with regard to the apparent discrepancy between the 50–150 nm periodicity of the recognition lines and the 25 nm periodicity of the topographic bands. Presumably, this feature is inherent to the AFM force spectroscopy technique. Indeed, the lateral resolution in force spectroscopy is ∼ 15 nm (pixel size), whereas topographic images have a resolution of 2–5 nm. As the pixel size in recognition images is on the order of band periodicity, we expect discrete parallel lines to be observed only at low binding frequency ( Fig. 6b–d ), thus low force, although they can no longer be discriminated at high binding frequency ( Fig. 6e ). Hence, resolving 25-nm-wide bands in recognition images would require improving the resolution by a factor of 5, which was technically not possible. Finally, to gain further insight into the peptidoglycan organization, we examined WPS − mutant cells using AFM tips functionalized with lectins. We used wheat germ agglutinin (WGA) and Griffonia simplicifolia lectin II (GSII) to probe peptidoglycan-associated N -acetylglucosamine (GlcNAc) residues, and non-reducing GlcNAc termini, respectively [11] . As shown in Supplementary Fig. S6 , we found that both WGA and GSII bound moderately and similarly to the surface of the VES5748 WPS − mutant. The recognition sites formed lines that were somewhat similar to those observed with the LysM tip but less defined, as indicated by the smaller R 2 values (0.75–0.9 versus 0.1–0.3 for randomly placed lines). The lack of differential binding between GSII and WGA suggests that non-reducing GlcNAc termini are not the main residues covering the cell surface. Our experiments show that AFM topographic and recognition imaging are complementary approaches to probe the nanoscale architecture of peptidoglycan in living Gram-positive bacteria. We provide several pieces of evidence which, in L. lactis , argue for an architectural feature in the plane perpendicular to the long axis of the cell ( Fig. 7 ) [11] , [39] . First, topographic images show that the surface of WPS − mutant strains lacking cell WPS displays 25-nm-wide periodic bands (ridges) running always parallel to the short cell axis. Second, analysis of a double mutant lacking both cell WPS and the major autolysin AcmA confirms that the observed ridges do not result from hydrolysis but are intrinsic features of the cell wall. Third, recognition imaging with LysM tips indicates that the observed bands are made of peptidoglycan, as peptidoglycan lines are found to run parallel to the short cell axis. Fourth, images of broken sacculi indicate that the cells generally fracture across their short axis, suggesting an architectural feature in this plane. As already pointed out for B. subtilis [11] , this orientated fracture plane is not consistent with the 'scaffold' model in which strands would be vertically oriented. 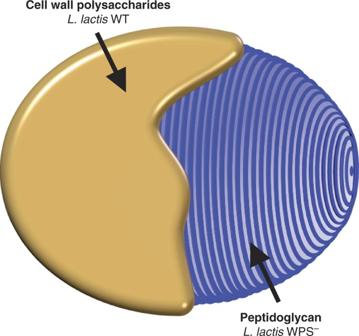Figure 7: Schematic drawing of the nanoscale organization of theL. lactispeptidoglycan. The cartoon emphasizes the outermost surface layers, that is, cell wall polysaccharides in WT cells, and peptidoglycan arranged as periodic bands in WPS−cells. Figure 7: Schematic drawing of the nanoscale organization of the L. lactis peptidoglycan. The cartoon emphasizes the outermost surface layers, that is, cell wall polysaccharides in WT cells, and peptidoglycan arranged as periodic bands in WPS − cells. Full size image Further experiments are needed to establish whether peptidoglycan bands reflect cables made of coiled bundles of glycan strands, such as in B. subtilis . In such a mechanism, glycan strands are polymerized and crosslinked to form a peptidoglycan 'rope', which is then coiled into a helical cable. It has been shown that peptidoglycan assembly relies on biosynthetic machineries that include penicillin-binding proteins (PBPs) associated with cytoskeleton proteins guiding the incorporation of newly synthesized peptidoglycan [40] , [41] . A challenging approach would be to apply AFM to bacteria combining mutations in genes encoding WPS and partners of biosynthetic machineries, such as PBPs and architectural MreCD proteins, or to examine WPS − mutant cells that are morphologically affected by β-lactam treatment that alters the function of one or more PBP(s). In summary, our study demonstrates that the combination of cell-envelope mutants with AFM is a powerful approach for analysing the nanoscale organization of bacterial cell walls. The use of mutant strains lacking outer cell wall layers is a valuable approach to reveal the organization of inner cell wall constituents directly in live cells, thus using neither any chemical or enzymatic treatment nor fixation or labelling procedures. Bacterial strains and growth conditions We used Lactococcus lactis strain NZ 3900 [42] as the WT, and strains VES5748 and VES5751 as exopolysaccharide (WPS) negative mutants [24] . Strain VES1876, carrying point mutation in gene llmg_0226 , leading to the WPS-negative phenotype, was isolated as resistant to the lactococcal bacteriophage sk1 derivative [24] from strain MG1363 acmA Δ1, carrying deletion of the main autolysin gene acmA [37] . These strains are derivatives of the model L. lactis strain MG1363 [43] . Bacteria were grown in M17 (Merck) medium supplemented with 1% glucose (Sigma) at 30 °C. For AFM analyses, bacteria were collected by centrifugation from exponentially growing cultures (optical density at 600 nm, OD 600 nm , of 0.3) and resuspended in acetate buffer (150 mM sodium acetate, pH 4.75), TrisMaleate buffer (50mM maleic acid, 40 mM Tris, pH 5.3), PBS (140 mM NaCl, 10 mM PO 4 buffer, 3 mM KCl, pH 7.4) or ultrapure water (Milli-Q, Millipore). AFM measurements AFM images and force–distance curves were recorded either in acetate buffer (imaging) or in TrisMaleate (force measurements), at room temperature, using a Nanoscope V Multimode AFM (Veeco Metrology Group). Sharpened silicon nitride cantilevers (MSCT, Veeco) and gold-coated cantilevers (OMCL-TR4, Olympus) were used for imaging and force measurements, respectively. Cells were immobilized by mechanical trapping into porous polycarbonate membranes (Millipore) with a pore size similar to the bacterial cell size [25] . After filtering a concentrated cell suspension, the filter was gently rinsed with the adapted buffer, carefully cut (1×1 cm) and attached to a steel sample puck (Veeco); the mounted sample was then transferred into the AFM liquid cell while avoiding dewetting. Statistical analysis of the width of the periodic features observed in the height images was performed by analysing multiple vertical cross-sections through the images. Unless otherwise stated, all force curves were recorded with a maximum applied force of ∼ 250 pN, with a loading rate of 13,000 pN s −1 . The spring constants of the cantilevers were measured using the thermal noise method (Picoforce, Veeco), yielding a mean value of 0.02 N m −1 . Adhesion force maps were obtained by recording 16×16 or 32×32 force–distance curves on areas of given size, calculating the adhesion force for each force curve and displaying the adhesion value as a grey pixel. For molecular recognition, recombinant AcmA cell wall-binding domains (kindly supplied by K. Leenhouts) [44] bearing a cysteine residue near the end of their N-terminal ends were immobilized onto gold-coated AFM tips. Before use, gold-coated cantilevers were cleaned for 15 min by ultraviolet/ozone treatment (Jelight), rinsed with ethanol and dried with a gentle nitrogen flow. They were immersed overnight in PBS solutions containing 10 μg ml −1 of recombinant peptide for 12 h, rinsed three times with buffer and briefly sonicated to remove aggregates that may be adsorbed. To prepare L. lactis sacculi, cells from exponential phase cultures were boiled in the presence of sodium dodecyl sulphate and next deproteinized by treatment with pronase and trypsin [45] . Nucleic acids were removed by DNAse and RNAse. Sacculi were then treated with trichloroacetic acid 10% to remove teichoic acids, and finally gently broken using a french press at a pressure of 500 psi. For AFM imaging, a drop of a diluted suspension of sacculi was deposited on freshly clived mica and air-dried. X-ray photoelectron spectroscopy WT and mutant cells were collected from exponentially growing cultures, resuspended in MilliQ water (Millipore) and directly lyophilized. XPS analyses were performed on a Kratos Axis Ultra spectrometer (Kratos Analytical) equipped with a monochromatized aluminium X-ray source. The angle between the normal to the sample surface and the electrostatic lens axis was 0°. The analysed area was ∼ 700×300 μm. The constant pass energy of the hemispherical analyser was set at 40 eV. The following sequence of spectra was recorded: survey spectrum, C 1s , N 1s , O 1s , P 2p , S 2p and C 1s again, to check the stability of charge compensation as a function of time and the absence of degradation of the sample during the analyses. To assess the level of surface contamination, sorbitol was included in the analyses, starting from the freeze-drying process. Binding energies were calculated with respect to the C -(C,H) component of the C1s peak of adventitious carbon fixed at 284.8 eV. Following subtraction of a linear baseline, molar fractions were calculated (CasaXPS program, Casa Software) using peak areas normalized on the basis of acquisition parameters, sensitivity factors and the transmission function provided by the manufacturer. Autolysis assays Bacteria from exponentially growing cultures were washed twice, resuspended in the relevant buffer and the optical density at 600 nm (OD 600 nm ) of the suspensions was measured every 20 min using a Varioskan Flash multimode reader (Thermo Scientific). How to cite this article: Andre, G. et al . Imaging the nanoscale organization of peptidoglycan in living Lactococcus lactis cells. Nat. Commun. 1:27 doi: 10.1038/ncomms1027 (2010).